Soft tissue preservation in a fossil marine lizard with a bilobed tail fin Mosasaurs are secondarily aquatic squamates that became the dominant marine reptiles in the Late Cretaceous about 98–66 million years ago. Although early members of the group possessed body shapes similar to extant monitor lizards, derived forms have traditionally been portrayed as long, sleek animals with broadened, yet ultimately tapering tails. Here we report an extraordinary mosasaur fossil from the Maastrichtian of Harrana in central Jordan, which preserves soft tissues, including high fidelity outlines of a caudal fluke and flippers. This specimen provides the first indisputable evidence that derived mosasaurs were propelled by hypocercal tail fins, a hypothesis that was previously based on comparative skeletal anatomy alone. Ecomorphological comparisons suggest that derived mosasaurs were similar to pelagic sharks in terms of swimming performance, a finding that significantly expands our understanding of the level of aquatic adaptation achieved by these seagoing lizards. Convergent evolution has resulted in some remarkable morphological adaptations in organisms that are found in similar environments. A classic example is the streamlined body shape and fluked tail developed by cetaceans and fish to allow swift movement through the water. Piscine body plans and bilobed caudal flukes have also been documented in two groups of distantly related Mesozoic marine reptiles; that is, ichthyosaurs and metriorhynchid crocodyliforms, thanks to rare soft tissue impressions in exceptionally preserved fossils [1] , [2] , [3] . However, to date, no similar soft tissue evidence has been reported in mosasaurs, despite a remarkably rich fossil record and a collection history that spans almost 250 years [4] . This lack of evidence, combined with conflicting hypotheses of the phylogenetic affinities of mosasaurs within Squamata [5] , [6] , [7] , [8] , [9] , have fuelled the cliché serpentine and lizard-like depictions of mosasaurs that dominate both the scientific and popular literature [10] , [11] , [12] , [13] . Moreover, studies of locomotor performance in mosasaurs have been hampered, because they have largely relied on incorrect descriptions and reconstructions of the derived mosasaur body plan (that is, a long, rectilinear body and straight, elongate tail). These errors in assumption have lead to the hypothesis that mosasaurs were slow-swimming animals capable of only short burst of speed during brief ambush pursuits [2] , [11] , [14] , [15] , [16] . Although early members of the group almost certainly utilized an undulating motion as a primary means of propulsion, the question remains how far the subsequent, better aquatically adapted forms came toward achieving a more energy-efficient, sustained swimming style. Fundamental to our understanding of mosasaur locomotion, and the degree of aquatic adaptation they achieved, is knowledge of the form, function and development of their tail flukes. Historically, the predominant view was that the fin-like extremity, of even derived mosasaurs, was virtually straight and spatulate, ‘like that of a great eel’ [17] . Reconstructions of crescent-shaped flukes were few [18] and were dismissed as being based on poorly preserved specimens [11] , or viewed as in conflict with existing skeletal evidence [10] , [11] . Nonetheless, over the last few years a growing body of data gathered from morphometric and comparative anatomical studies have indicated that the distal third of the mosasaur tail was structurally downturned in life and, in that regard, was similar to the hypocercal caudal flukes of derived ichthyosaurs and metriorhynchid crocodyliforms [19] , [20] , [21] , [22] , [23] . It has even been suggested [21] , [22] , [23] that certain advanced forms had semilunate tails resembling those of pelagic sharks (although dorsoventrally mirrored), but until now no soft tissue evidence to support these claims has been reported. Here we describe an exquisitely preserved specimen (ERMNH HFV 197; Eternal River Museum of Natural History) of a small-sized mosasaurine mosasaur from the Upper Cretaceous (Maastrichtian) Konservat-Lagerstätte of Harrana in central Jordan. The fossil has been mentioned previously in an abstract [24] and its skeletal morphology has been generally examined in a book chapter [25] . Here, however, we report the full preparation of ERMNH HFV 197, including unique details of its soft tissue anatomy. In addition to being largely articulated and complete from the fifth cervical vertebra to the distal fourth of the caudal segment, the fossil preserves in great fidelity a gentle ventral tailbend and large portions of integument, revealing, for the first time in a mosasaur, the soft tissue outline of a tail fin. ERMNH HFV 197 provides definitive evidence that derived mosasaurines were propelled by bilobed, asymmetrical caudal flukes, to demonstrate that mosasaurs are convergent with ichthyosaurs, metriorhynchid crocodyliforms and whales in the development of a specialized, crescent-shaped propulsive surface for enhanced locomotor efficiency. Geological context and age The specimen comes from the Muwaqqar Chalk Marl Formation (MCMF), which is part of the Belqa Group, and spans the Cretaceous/Paleogene boundary. The sediments were deposited on the southern margin of the Neo-Tethys Ocean [26] . The strata comprise mainly chalk and locally bituminous chalky marl with abundant limestone and chert concretions, and have been interpreted as a deep-water pelagic deposit [26] . The MCMF is part of a larger Upper Cretaceous–Eocene carbonate and phosphate sequence that extends across northern Africa and into the Middle East [27] . Phosphatic deposits formed in areas of high primary productivity are known to preserve abundant vertebrate fossils, including remains of, for example, mosasaurs, plesiosaurs, sharks, bony fish, turtles and marine crocodylians [27] , [28] . With the notable exception of ref. 25 , reports of Cretaceous vertebrates from the phosphatic deposits of Jordan have hitherto been based on a relatively limited material; however, the fossils indicate a diverse fauna similar in composition to that of Morocco [28] , [29] , [30] , [31] . On the basis of sequence stratigraphy [26] and microfaunal composition [32] , the oldest fossils from the MCMF are early to mid-Maastrichtian in age, although the age of the remaining Cretaceous part of the formation is unknown (including its precise age in the Harrana area and whether or not it reaches the Cretaceous/Paleogene boundary). The specimen ERMNH HFV 197 was collected in 2008 from a single micritic limestone concretion by one of us (HFK). The specimen has been cleaved along the sagittal plane and is disposed on two main slabs (collectively registered as ERMNH HFV 197-A) and a counterpart (ERMNH HFV 197-B), displaying a largely articulated mosasaur skeleton that is complete, save for the head and distal fourth of the tail ( Fig. 1 ). The bones are generally in a pristine condition and retain their original three-dimensional shape, although some skeletal elements were fractured or lost during the excavation of the fossil; the latter are now represented by natural moulds. In addition, plant rootlets have penetrated and partially dissolved a string of vertebrae near the end of the tail. The exposed elements of the pectoral girdle and rib cage are somewhat disturbed and the latter structure has suffered slight crushing; otherwise, the skeleton is in nearly perfect articulation, preserving, for example, a virtually complete, hydrofoil-like forelimb surrounded by skin impressions ( Figs 1 and 2 ) and the original configuration of the fan-like structure formed by the neural spines in the posteriormost intermediate caudal and terminal caudal series ( Figs 1 and 3a,b ). 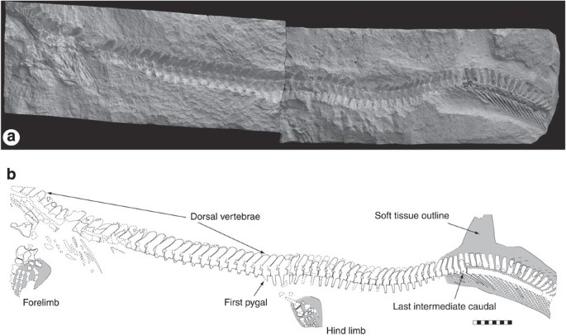Figure 1:Prognathodonsp. ERMNH HFV 197-A from the Maastrichtian MCMF of Harrana. (a) Photograph and (b) sketch indicating the bones and different skin structures preserved. Note that the soft tissue outline of the paddles and caudal fin is readily visible, whereas the body is represented by skeletal elements alone (with the possible exception of a purple-reddish stain located within the chest cavity). Scale bar, 10 cm. Figure 1: Prognathodon sp. ERMNH HFV 197-A from the Maastrichtian MCMF of Harrana. ( a ) Photograph and ( b ) sketch indicating the bones and different skin structures preserved. Note that the soft tissue outline of the paddles and caudal fin is readily visible, whereas the body is represented by skeletal elements alone (with the possible exception of a purple-reddish stain located within the chest cavity). Scale bar, 10 cm. 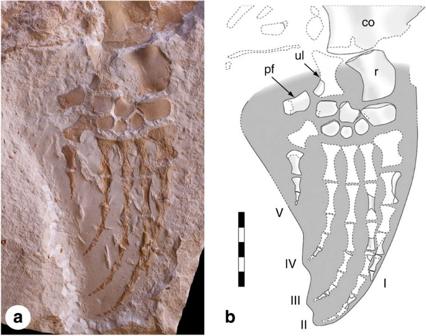Figure 2: Left forelimb ofPrognathodonsp. ERMNH HFV 197-B in medial view. (a) Photograph and (b) interpretative drawing. Note near-perfect articulation of skeletal elements and virtually intact outline of soft tissues. Note also how the position of the pisiform expands the fin surface and how the anterior digits intimately follow the leading edge of the paddle, thereby contributing to a semi-streamlined parasagittal profile similar to that of sectioned ichthyosaur and porpoise fins (cf. ref.60). Scale bar, 5 cm. co, coracoid; pf, pisiform; r, radius; ul, ulna; I–V, digits 1–5. Full size image Figure 2: Left forelimb of Prognathodon sp. ERMNH HFV 197-B in medial view. ( a ) Photograph and ( b ) interpretative drawing. Note near-perfect articulation of skeletal elements and virtually intact outline of soft tissues. Note also how the position of the pisiform expands the fin surface and how the anterior digits intimately follow the leading edge of the paddle, thereby contributing to a semi-streamlined parasagittal profile similar to that of sectioned ichthyosaur and porpoise fins ( cf . ref. 60 ). Scale bar, 5 cm. co, coracoid; pf, pisiform; r, radius; ul, ulna; I–V, digits 1–5. 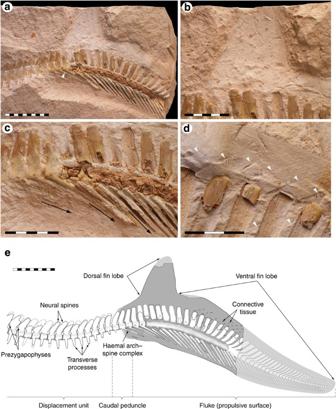Figure 3:Prognathodonsp. ERMNH HFV 197-A tail fluke with soft tissues. (a) An overview of the caudal region preserving the tail fin. Note that the downturned section of the caudal skeleton lacks transverse processes (the last intermediate caudal is marked with an arrowhead), to suggest that the fluke was laterally flattened. (b) A close-up of the fleshy dorsal fin lobe. Note how the neural spines change in orientation along the depicted vertebral section, forming a vertically dilated, fan-like extremity. (c) Close-up of the vertebrae at the base of the expanded portion of the tail. Arrows indicate the changing inclination of the fused chevrons of the haemal arch–spine complexes at the transition from intermediate to terminal caudal vertebrae, representing their original configuration. (d) Connective tissue (arrowheads) and its relationship to the spinous processes of the vertebrae in the ventral fin lobe. In addition to contributing to a streamlined cross-section, the inclination of the fibrous structures suggests that they served to stiffen the fluke during its sideways excursions. (e) Reconstructed tail fin ofPrognathodonsp. Whereas the tip of the dorsal fin lobe was confidently reconstructed from a photograph taken during the excavation of ERMNH HFV 197, the distalmost portion of the tail is based on the caudal skeleton of the closely related mosasaurineClidastes propython(KUVP 1022; Natural History Museum and Biodiversity Research Center). The number of missing vertebrae was estimated by visual comparison and interpolation of dimensional data. Scale bars, (a,e) 10 cm, (b,c) 5 cm and (d) 3 cm. Full size image Figure 3: Prognathodon sp. ERMNH HFV 197-A tail fluke with soft tissues. ( a ) An overview of the caudal region preserving the tail fin. Note that the downturned section of the caudal skeleton lacks transverse processes (the last intermediate caudal is marked with an arrowhead), to suggest that the fluke was laterally flattened. ( b ) A close-up of the fleshy dorsal fin lobe. Note how the neural spines change in orientation along the depicted vertebral section, forming a vertically dilated, fan-like extremity. ( c ) Close-up of the vertebrae at the base of the expanded portion of the tail. Arrows indicate the changing inclination of the fused chevrons of the haemal arch–spine complexes at the transition from intermediate to terminal caudal vertebrae, representing their original configuration. ( d ) Connective tissue (arrowheads) and its relationship to the spinous processes of the vertebrae in the ventral fin lobe. In addition to contributing to a streamlined cross-section, the inclination of the fibrous structures suggests that they served to stiffen the fluke during its sideways excursions. ( e ) Reconstructed tail fin of Prognathodon sp. Whereas the tip of the dorsal fin lobe was confidently reconstructed from a photograph taken during the excavation of ERMNH HFV 197, the distalmost portion of the tail is based on the caudal skeleton of the closely related mosasaurine Clidastes propython (KUVP 1022; Natural History Museum and Biodiversity Research Center). The number of missing vertebrae was estimated by visual comparison and interpolation of dimensional data. Scale bars, ( a , e ) 10 cm, ( b , c ) 5 cm and ( d ) 3 cm. Full size image Taxonomy ERMNH HFV 197 was originally described in 2009 and was designated as the holotype of Tenerasaurus (from Tenera , La., young or immature; sauros , Gr., lizard) hashimi in recognition of its small size (as preserved, ~1.5 m in length) and presumed juvenile ontogenetic stage [25] . Within Mosasauridae, possession of fused haemal arch–spine complexes supports referral to the subfamily Mosasaurinae [6] . The skeletal anatomy of Tenerasaurus agrees in all observable respects with the generic diagnosis of the genus Prognathodon [33] and is therefore referred to that taxon here. This taxonomic reassignment is also supported by the fact that Prognathodon is represented by numerous larger individuals in the MCMF [25] and more broadly in the Middle East and Africa [34] , [35] . Discovery of soft tissues During examination of ERMNH HFV 197 in December 2011, the senior author (JL) discovered what appeared to be soft tissue remains surrounding the distalmost portion of the caudal vertebral column. This prompted a re-investigation of the fossil with the aim of exposing further skin structures that may still be hidden in the matrix, and over the course of two days the tail of ERMNH HFV 197 was prepared using small chisels and a pneumatic microscribe. This action uncovered significant parts of a bilobed fluke preserved as a thin, buff-coloured film ( Figs 1 and 3 ); however, the fragile nature of the skeleton and the presence of uranium minerals in intimate association with the bones discouraged preparation beyond the posteriormost intermediate caudals. Nonetheless, close inspection of the matrix surrounding the dorsal edge of the vertebral column did not reveal any putative skin structures or soft tissue impressions anterior to the expanded fin-like extremity. Furthermore, it was readily apparent that the tip of the dorsal fin lobe of the caudal fluke had been lost during the initial preparation of the specimen before the recognition that soft tissues were preserved. An accurate reconstruction ( Fig. 3e ) was possible, however, on the basis of a photograph taken in the field during the excavation of ERMNH HFV 197, in which the apex of the dorsal fin lobe was visible on the exposed bedding surface of the freshly split concretion. Description of caudal skeleton Notwithstanding breakage of numerous vertebral processes (which are represented by natural moulds), the caudal segment of the vertebral column of ERMNH HFV 197 is reasonably complete, comprising a consecutive series of at least six pygals (the confirmed, minimum count), 23 intermediate caudals and 17 terminals. On the basis of the known caudal vertebral counts in the closely related mosasaurines Clidastes and Mosasaurus [5] , [23] , the estimated original number of terminals in ERMNH HFV 197 is confidently predicted at 47, resulting in a total caudal vertebral count of 76. The vertebrae at the base of the caudal series (that is, the pygals) are almost identical to the posteriormost dorsals; in which, the centra are cylindrical, functional zygapophyses are present and the neural spines are in the form of semi-rectangular plates that slope backward at a similar angle ( Fig. 1 ). However, contrary to the preceding dorsals that hold stubby synapophyses, the pygals bear long, ventrolaterally projecting transverse processes. Posteriorly along the intermediate caudal series, the central bodies decrease progressively in length, and the zygapophyseal contacts between successive vertebrae are gradually lost (although vestigial prezygapophyses occur through the greater part of the intermediate caudal segment). As the vertebrae become shorter, the transverse processes diminish in size, and towards the distal end of the intermediate caudal series they also begin a gradual rise on the centra, culminating in rudimentary outgrowths located some distance from the ventrolateral edges of the centrum of the last intermediate caudal vertebra ( Fig. 3a , arrowhead). The neural spines assume a relatively slender lateral outline and upright orientation in the proximal intermediate caudal section ( Fig. 1 ), only to resume a posterior inclination and constant, gradual decrease in height further rearward ( Figs 1 and 3a,e ). These vertebral processes regain their height once again, however, and become progressively more erect in the posteriormost portion of the intermediate caudal series. On the last intermediate caudal vertebra, the neural spine is greatly elongated and almost perpendicular to the long axis of the centrum. Further posteriorly, the neural spines become increasingly anteriorly inclined until the fourth terminal caudal vertebra, and although still projected anteriorly they gradually become less so until the eighth terminal, forming a conspicuous arcuate fringe ( Figs 1 and 3a,b,e ). Behind this expanded region, the neural spines are strongly posteriorly inclined near the base, but become more vertically oriented distally. Fused chevrons of the haemal arch–spine complexes are only visible near the preserved distal end of the tail, and in the accessible section they change from being gently ventroposteriorly inclined (at about 20° to the long axis of the corresponding centra) on the last intermediate caudals to progressively more vertically oriented on the anteriormost terminals ( Fig. 3c , arrows). From the third terminal caudal vertebra, the chevrons slope uniformly backward at an angle of about 35° to the horizontal vertebral axis. These morphological changes are accompanied by a gentle structural flexure of the entire caudal vertebral column of ERMNH HFV 197, producing a slight dorsal bend anterior to a more significant ventral displacement ( Figs 1 and 3a,e ). Given that the tails of derived mosasaurine mosasaurs partially comprise dorsally wedge-shaped vertebrae (vertebrae where the dorsal centrum edge is longer than the ventral centrum edge), and that the ratios of dorsal centrum length to ventral centrum length peak in the anterior terminal caudal series (that is, in the area showing the maximum flexure in ERMNH HFV 197) [19] , [20] , [21] , [22] , [23] , the downward bend produced by the posterior tail segment in ERMNH HFV 197 is here considered to represent the natural condition. However, the preceding upward curvature is probably artificial, as indicated by the shifting directions of the transverse processes and partially overlapping neural spines ( cf . ref. 22 ). Description of soft tissues The soft tissues associated with the distal portion of the caudal vertebral segment are preserved as a buff-whitish film, which forms a bedding-parallel surface that easily separates from the surrounding concretion. Scanning electron microscopic–energy-dispersive X-ray point sum spectrum analysis revealed distinct peaks in calcium and oxygen ( Fig. 4 ), suggesting that the buff material primarily comprises calcium carbonate. Faint, rhomboidal scale impressions are present along the trailing edge of the dorsal fin lobe and above the neural spines in the ventral fin lobe ( Fig. 5 ). The outline of the preserved soft tissues defines in great fidelity the asymmetric bilobed planform shape of the caudal fluke ( Fig. 3 ). Whereas the ventral fin lobe closely follows the downturned vertebral column, the unsupported dorsal fin lobe forms a distally tapering, wing-like structure above the arcuate extremity formed by the neural spines at the intermediate/terminal caudal vertebral transition ( Fig. 3b,e ). The leading edge of the dorsal fin lobe is gently convex, distinctly rearward inclined and somewhat longer than the slightly anteriorly oriented trailing edge. 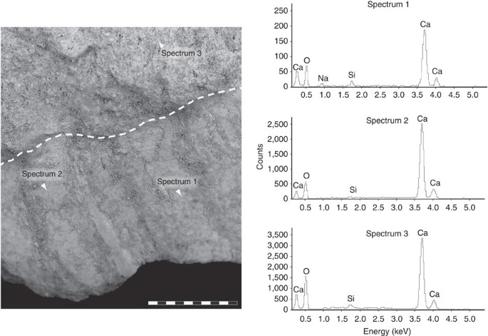Figure 4: Scanning electron microscopic–energy-dispersive X-ray analysis of fossil skin (Spectrum 1 and 2) and sediment (Spectrum 3). Note distinct peaks in calcium (Ca) and oxygen (O) in all three spectra, suggesting that both the integument and sediment primary comprise calcium carbonate. The dashed line demarcates skin replacement structures (bottom) and sedimentary matrix (top). Scale bar, 1 mm. Figure 4: Scanning electron microscopic–energy-dispersive X-ray analysis of fossil skin (Spectrum 1 and 2) and sediment (Spectrum 3). Note distinct peaks in calcium (Ca) and oxygen (O) in all three spectra, suggesting that both the integument and sediment primary comprise calcium carbonate. The dashed line demarcates skin replacement structures (bottom) and sedimentary matrix (top). Scale bar, 1 mm. 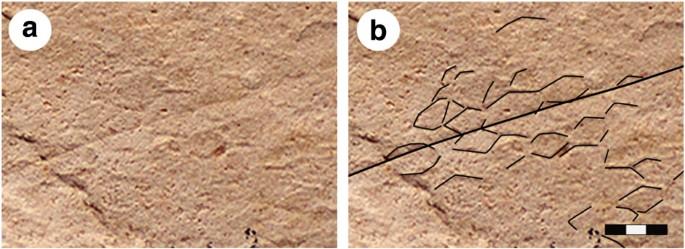Figure 5: Integumentary structures ofPrognathodonsp. ERMNH HFV 197-A. (a) Imprints of articulated scales and connective tissue above the vertebral column in the ventral fin lobe ofPrognathodonsp. (b) Same photograph as ina, with outlines of preserved scale impressions. Measurable scales range from about 1.0 to 1.5 mm in height and 1.5 to 2.0 mm in length. Scale bar, 3 mm. Full size image Figure 5: Integumentary structures of Prognathodon sp. ERMNH HFV 197-A. ( a ) Imprints of articulated scales and connective tissue above the vertebral column in the ventral fin lobe of Prognathodon sp. ( b ) Same photograph as in a , with outlines of preserved scale impressions. Measurable scales range from about 1.0 to 1.5 mm in height and 1.5 to 2.0 mm in length. Scale bar, 3 mm. Full size image Only the proximal half of the ventral fin lobe is preserved. The buff-coloured film reveals that the soft tissues originally extended well beyond the caudal skeleton dorsally ( Fig. 3d,e ); however, on the ventral side the film terminates a short distance beyond the distal ends of the fused chevrons of the haemal arch–spine complexes ( Fig. 3a,e ). Thus, judging from the relationship between the axial skeleton and soft tissues, the ventral fin lobe must have had a streamlined cross-section with a blunt leading edge and a tapering trailing edge. Weak impressions of fibrous structures that slope regularly rearward at about 30° to the long axis of the vertebral column occur dorsally and laterally to the neural spines in the fluke area ( Fig. 3d , arrowheads), to suggest that thick sheets of connective tissue once straddled the spinous processes in the ventral fin lobe. Similar to most fish and cetaceans, mosasaurs are considered axial swimmers in that, they generated propulsive thrust by means of bodily and caudal fin undulations, while the flippers were primarily used as steering devices [5] , [14] , [15] , [21] , [22] , [23] , [36] . On the basis of regional variations in vertebral centrum dimensions and discrepancies in vertebral process length and orientation, Lindgren et al . [21] , [22] , [23] divided the caudal vertebral column of derived mosasaurs into four discrete subunits, including: (1) a proximal tail stock, formed by the tallest and widest vertebral centra; that is, the pygals, which acted as a reinforced foundation upon which the undulations took place; (2) a mid-sectional displacement unit, formed by the greater part of the intermediate caudal series, which swept from one side to the other; (3) a narrow caudal peduncle, identified by vertebrae with relatively short neural spines and ventroposteriorly inclined haemal arch–spine complexes, which cut through the water with minimal resistance; and (4) a distal propulsive surface ( Fig. 3e ). Furthermore, based on comparisons with the skeletal and fin structures of modern sharks, Lindgren et al . [21] , [22] , [23] hypothesized that mosasaurs, in fact, not only had a downturned tail forming a ventral fin lobe but also possessed a fleshy dorsal fin lobe, together forming an asymmetric hypocercal tail fluke. That prediction is verified by the preserved soft tissues in ERMNH HFV 197. Given that the tail fluke represents the distalmost portion of the vertebral axis, and thus is the place where water accelerated posteriorly leaves the body, its shape dramatically influences performance in axial-undulatory swimming animals [37] , [38] , [39] . For instance, the tail fin of ERMNH HFV 197 shows a number of features for improved efficiency by reduced induced drag, including the backward-curved leading edge and virtually straight trailing edge of the dorsal fin lobe. Steady-flow theory [40] predicts that this shape provides a 4.5% increase in induced efficiency compared with a similar-sized fin with an elliptical planform. Furthermore, the inferred streamlined sectional profile of the ventral fin lobe formed by the anteroventrally located vertebral column and dorsal plate of connective tissue would have provided enhanced lift for thrust, while minimizing induced drag ( cf . ref. 41 ). The dorsal connective tissues would not only have contributed to a tapering trailing edge, but also to enhanced stiffness through the oblique inclination of the individual fibre bundles ( Fig. 3d ), an arrangement that would have allowed the construction of a rigid propulsive surface to thrust effectively against the water. The proportions of the soft tissue structures and their relationship with the skeletal elements in ERMNH HFV 197 provide an empirical basis for reconstructions of fin outlines in other specimens, although this must be approached with caution. ERMNH HFV 197 is conspicuously small by Prognathodon standards, a genus in which adult individuals sometime exceed 10 m in body length [33] . Therefore, ERMNH HFV 197 is here assumed to represent a juvenile animal. Positive allometric tail fin growth with body size has been documented in, for example, ichthyosaurs and the great white shark, Carcharodon carcharias [42] , [43] , [44] . This enlargement is driven by the increased demand on the amount of thrust generated by the propulsive organ as mass and surface area of the animal increase. Most previous investigations have focused on forms possessing a symmetrical lunate tail fluke, unlike that in mosasaurs. However, in a study of ontogenetic shape change in the spiny dogfish shark, Squalus acanthias (a form that possesses an asymmetric tail fin), allometric scaling of the caudal fin span versus body length was also detected (manifested as an elongated and narrowed dorsal fin lobe and a broadened and ventrally expanded ventral fin lobe in larger individuals) [45] . Therefore, it is likely that larger individuals of Prognathodon would have had a proportionally larger caudal fin relative to the body length, with a relatively larger dorsal fin lobe than that preserved in the presumed juvenile specimen reported here. How this relates to other mosasaurs is less clear; however, we can say with confidence that the osteological correlates of a tail fluke, as previously documented [21] , [22] , [23] , can be used to justify placement, if not proportion, of the dorsal fin lobe in derived mosasaurs. Extant steady swimmers have independently evolved streamlined bodies that are propelled by forked caudal fins mounted on slender tail sections, as seen in pelagic fish, sharks and cetaceans [37] , [46] , [47] . This morphological configuration optimizes locomotor efficiency while reducing pressure drag [40] , [43] , [48] , whereas the diversity in body design that exists within this general framework among modern cruisers reflects compromises needed to balance requirements for speed, acceleration, efficiency and manoeuvrability [47] , [49] . It has previously been shown that different modes of undulatory locomotion can generally be correlated with different body shapes [50] , and the relationship between swimming performance and body form has been examined using both empirical and numerical methods [38] , [39] . However, the morphology of the asymmetric tail fin in mosasaurs falls between the two categories previously examined [38] , [39] , and no numerical studies of hypocercal (or epicercal) performance in various kinematic regimes are available, although a recent investigation of tail form employing passive robotic swimmers did include epicercal variants in the form of foils with an angled trailing edge [51] . These epicercal foils yielded higher velocities for any given tail beat frequency, but were found to be less efficient in terms of power requirements. Although numerical modelling of the performance characteristics of hypocercal tails in free swimming experiments would be valuable to show in a quantitative way the specific effects of variation in fin configuration, some insights can be gained by comparing mosasaurs with sharks in terms of body form and potential swimming characteristics. The tail fin of ERMNH HFV 197 is clearly asymmetric ( Fig. 3e ) and, as such, has a planform shape similar to those of carcharhinid sharks, albeit being turned upside down ( cf . ref. 46 ). However, the superficial similarity between sharks and derived mosasaurs is not limited to their caudal flukes, but is also readily apparent in the streamlined shape of their bodies. An anterior migration of the long ribs (that is, those attached to the sternum and anterior dorsal vertebrae) has been known in mosasaurs for some time [5] . Accompanying this migration is a forward shifting of the abdominal viscera, documented in an exceptionally preserved specimen (LACM 128319; Natural History Museum of Los Angeles County) of the russellosaurine mosasaur Platecarpus [22] , [52] . Judging from the flattened but otherwise virtually intact rib cage of ERMNH HFV 197, and with additional data/measurements taken from the closely related mosasaurines Prognathodon overtoni [33] and Prognathodon saturator [53] , it is clear that at least in these relatively derived mosasaurs, the anterior body was fairly deep, but quickly narrowed posteriorly, reaching its narrowest point just anterior to the tail fluke ( Fig. 6a ). 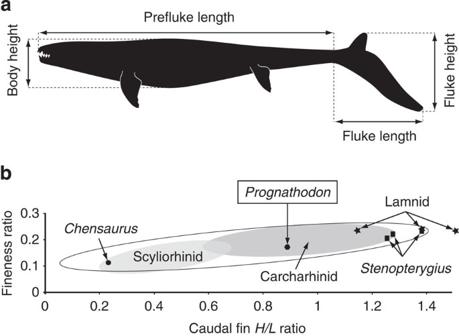Figure 6: Reconstructed profile of ERMNH HFV 197 and body shape correlation between taxa. (a) Hypothetical body outline ofPrognathodonbased on ERMNH HFV 197 with added data/measurements fromP.overtoniandP.saturator. Note that the artificial dorsal tail curvature produced by the pygal and anterior intermediate caudal vertebrae in ERMNH HFV 197 has been eliminated (based on a comparison with the virtually intact and articulated tail of LACM 128319 (refs22,52)), resulting in a deeper caudal fin with a higher aspect ratio. (b) Body and tail form distribution in modern scyliorhinid, carcharhinid and lamnid sharks, two Mesozoic ichthyosaurs (ChensaurusandStenopterygius) andPrognathodon. The diagram in is redrawn from ref.55with added data from ERMNH HFV 197. Figure 6: Reconstructed profile of ERMNH HFV 197 and body shape correlation between taxa. ( a ) Hypothetical body outline of Prognathodon based on ERMNH HFV 197 with added data/measurements from P . overtoni and P . saturator . Note that the artificial dorsal tail curvature produced by the pygal and anterior intermediate caudal vertebrae in ERMNH HFV 197 has been eliminated (based on a comparison with the virtually intact and articulated tail of LACM 128319 (refs 22 , 52 )), resulting in a deeper caudal fin with a higher aspect ratio. ( b ) Body and tail form distribution in modern scyliorhinid, carcharhinid and lamnid sharks, two Mesozoic ichthyosaurs ( Chensaurus and Stenopterygius ) and Prognathodon . The diagram in is redrawn from ref. 55 with added data from ERMNH HFV 197. Full size image Because of the asymmetry present in the tail fin, there is the obvious question of how thrust was produced (it would appear to have had a significant posteroventral component), and how that thrust was translated into forward motion. In a model dealing with the mechanics of the epicercal tail fin of sharks [54] , the forward thrust vector passes through the centre of gravity by balancing the posteroventral thrust generation (along the heterocercal angle) with offsetting thrust generated by the rotational attitude of the trailing edge of the dorsal fin lobe. The forces generated by the ventral fin lobe are produced in a similar fashion, but as this lobe is offsetting some of the forces of the dorsal fin lobe, it also acts to reduce the effective thrust angle. Interestingly, it has been concluded [46] that a ventral fin lobe is a ‘necessity’ in all cases where the heterocercal angle exceeds 33°, and ‘would be extremely useful at lower ranges, say 15° to 26°, because it would reduce the angle of rotation needed for ‘balance’’. In mosasaurs, of course, the fin lobes are reversed, the ventral one being the primary thrust generator, but together with the dorsal fin lobe, presumably behaved in a way similar to those in sharks. In fact, the ventral fin lobe of the tail fluke in ERMNH HFV 197 approaches 33°; thus, the presence of a dorsal fin lobe is predicted in ref. 46 . Notwithstanding other differences in the body form of mosasaurs when compared with that of sharks (for example, centre of balance, placement and size of the front and hind fins, and shape of the head), it would appear that sharks may be a reasonable living analogue to infer, at least broadly, the locomotor performance of mosasaurs, as employed by Motani et al . [55] in a study of ichthyosaur swimming styles. Using basic indices, such as fineness ratio (body height/prefluke length; Fig. 6a ) and tail H / L (fluke height/fluke length), to quantify variation in body and tail shape among sharks and ichthyosaurs, Motani et al . [55] were able to demonstrate that basal ichthyosaurs, such as Chensaurus ( Fig. 6b ), had body proportions similar to those of scyliorhinid sharks, and hence presumably utilized anguilliform modes of swimming (that is, large parts of their bodies were thrown into undulations during locomotion). Conversely, highly derived taxa, such as Stenopterygius ( Fig. 6b ), grouped with lamnid sharks, which are known to be thunniform swimmers (that is, motion is restricted to the tail fin, whereas the body is held somewhat rigid during locomotion). When plotting data (see ref. 55 for method) from ERMNH HFV 197 onto this diagram ( Fig. 6b ), this mosasaur lies close to the centre of the carcharhinid distribution, to suggest that it may have had similar swimming performance characteristics as these sharks. The findings in the present study on the caudal fluke morphology of Prognathodon , along with recent previous work on the streamlined body shape [21] , [22] , [52] , keeled scales [56] and modified limbs [57] provide compelling evidence that derived mosasaurs were hydrodynamically advanced animals capable of high-efficiency swimming. Moreover, the emerging evidence suggests that aquatic adaptations evolved relatively quickly within the group (that is, within less than 10 million years [22] ) and likely convergently as well [23] , [58] , [59] . In addition, ERMNH HFV 197 demonstrates remarkable convergent evolution of body form with both fossil and extant marine amniotes, illuminating the relatively narrow adaptive corridor that these animals shared with their ecological brethren. The broad implications of these new data points are that convergent evolution is more common than suspected, and underscores the importance of recognizing the role of homoplasy in phylogentic analyses of long-lived, taxonomically diverse groups, such as mosasaurs, as it can easily remain hidden within the received wisdom of long held phylogenetic hypotheses. Scanning electron microscopy Samples selected for scanning electron microscopic analysis were mounted on glass slides using double-sided carbon tape. The screening was performed using a Hitachi S-3400N scanning electron microscope on uncoated samples under low vacuum, and the elemental composition was determined using energy-dispersive X-ray microanalysis (60 s analysis time at 15 keV, 62.0 μA and a working distance of 10 mm). How to cite this article: Lindgren, J. et al . Soft tissue preservation in a fossil marine lizard with a bilobed tail fin. Nat. Commun. 4:2423 doi: 10.1038/ncomms3423 (2013).